Mechanism of resilin elasticity Resilin is critical in the flight and jumping systems of insects as a polymeric rubber-like protein with outstanding elasticity. However, insight into the underlying molecular mechanisms responsible for resilin elasticity remains undefined. Here we report the structure and function of resilin from Drosophila CG15920. A reversible beta-turn transition was identified in the peptide encoded by exon III and for full-length resilin during energy input and release, features that correlate to the rapid deformation of resilin during functions in vivo . Micellar structures and nanoporous patterns formed after beta-turn structures were present via changes in either the thermal or the mechanical inputs. A model is proposed to explain the super elasticity and energy conversion mechanisms of resilin, providing important insight into structure–function relationships for this protein. Furthermore, this model offers a view of elastomeric proteins in general where beta-turn-related structures serve as fundamental units of the structure and elasticity. Resilin functions as a 'super elastic rubber' in specialized cuticle regions of most insects where extension and retraction are needed millions of times over the lifetime of the animals [1] . Naturally, crosslinked resilin exhibits high resilience, large strain and low moduli. Detailed mechanical characterisation demonstrated that the rubber-like protein had up to 95% resilience under high-frequency conditions [2] . It could be stretched to over 300% of its original length before breaking with low elastic modulus in the range of 0.1–3 MPa as indicated by scanning probe microscopy and tensile testing [3] . As to the unique mechanical properties of resilin, several studies have been reported to understand the relationships between structure and function of this protein system, as well as providing options for potential applications for biomaterials with super elasticity [4] , [5] . For example, a partial clone of resilin (rec1-resilin), from the first exon of Drosophila melanogaster , provided the major source of elasticity via unstructured amorphous features [3] , [6] . This rec1-resilin was not sufficient to store energy for jumping or flying of insects and must act as constituent of a composite with other domains in the resilin, such as the chitin-binding domain [5] , [7] . This result suggested a clue that the full-length resilin may function in both elasticity and energy storage. However, the mechanisms responsible for the storage of elastic potential energy in response to external stress remain unclear. Full-length resilin in D. melanogaster contains three significant domains ( Fig. 1 ): the first exon with 323 amino acids (exon I reported as 'pro-resilin'), comprising 18 pentadecapeptide repeats (GGRPSDSYGAPGGGN) [3] , [7] ; the second exon with 62 amino acids (exon II) determined to be a typical cuticular chitin-binding domain [7] , [8] ; and the third exon with 235 amino acids (exon III), comprising 11 tridecapeptide repeats (GYSGGRPGGQDLG) [8] . Despite progress in experimental and theoretical studies, thus far no model has been developed to enable a comprehensive understanding of the role of the two fundamental constituents derived from exon I and III of full-length resilin (that is, the resilin fibril nanostructure as shown in Fig. 1a ). This progress has partly been hindered due to a lack of a thorough understanding of the molecular mechanism for resilin elasticity at the nanoscale. 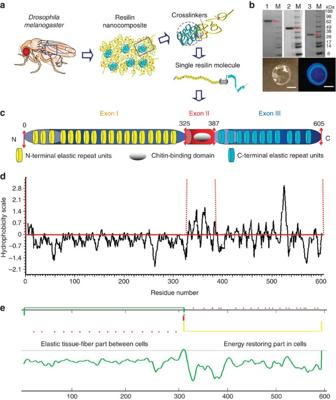Figure 1: Primary sequence and structure model of resilin inD. melanogaster. (a) Hierarchical structure of fruit fly resilin. The resilin fibrils with crosslinking consist of two major unstructured peptides derived from exon I and III of full-length resilin. (b) In total, 4–12% SDS–polyacrylamide gel electrophoresis of full-length resilin (lane 1), exon I (lane 2) and exon III (lane 3) samples from purification (upper panel) and fluorescence of full-length resilin film under white (left) and ultraviolet (right) light (lower panel). The scale bar is 5 mm. Seeblue plus2 pre-stained standard (Invitrogen, CA, USA) was used as size markers. (c) Amino-acid sequence scheme of three exons in the full-length resilin protein. (d) Hydrophobicity index of the full-length resilin. (e) Proposed transmembrane segment of resilin34. Figure 1: Primary sequence and structure model of resilin in D. melanogaster . ( a ) Hierarchical structure of fruit fly resilin. The resilin fibrils with crosslinking consist of two major unstructured peptides derived from exon I and III of full-length resilin. ( b ) In total, 4–12% SDS–polyacrylamide gel electrophoresis of full-length resilin (lane 1), exon I (lane 2) and exon III (lane 3) samples from purification (upper panel) and fluorescence of full-length resilin film under white (left) and ultraviolet (right) light (lower panel). The scale bar is 5 mm. Seeblue plus2 pre-stained standard (Invitrogen, CA, USA) was used as size markers. ( c ) Amino-acid sequence scheme of three exons in the full-length resilin protein. ( d ) Hydrophobicity index of the full-length resilin. ( e ) Proposed transmembrane segment of resilin [34] . Full size image Recently, we cloned and expressed the recombinant full-length resilin as a soluble protein in Escherichia coli [7] . To probe the molecular mechanism of resilin elasticity, we also produced the individual exon I and III polypeptides of resilin with a similar cloning strategy ( Fig. 1b , upper panel). Furthermore, we have previously shown that a similar fluorescence signature was confirmed for full-length resilin as previously reported for pro-resilin ( Fig. 1b , lower panel) [3] . In this paper, a new mechanistic model was developed to describe the elastic mechanisms of resilin, with contributions from the individual protein domains towards the behaviour of the full-length protein. Thermal treatments and thermal transitions Temperature-modulated differential scanning calorimetry (TM-DSC) techniques were first performed to measure the transition temperatures for the full-length resilin, exon I and III samples ( Fig. 2a ). The results indicated a two-step transition in the bound water-resilin system. A sharp endotherm around 50 °C was observed in the first transition, indicating a secondary or tertiary conformation change, perhaps like a helix-coil transition, which was found only in the peptides encoded by the two exons but not in the full-length resilin. This difference indicated a specific three-dimensional functional conformation for bound water in both exons with a quick 'melting' or 'relaxation' behaviour. After this step, the bound water molecules start to evaporate above 65 °C, shown as a broad endothermal peak in the heat capacity. Bound water was fully lost above 150 °C until the second transition for pure resilin starts at 201 °C. Finally, the resilin samples degrade above 250 °C. The total and reversing heat flow of TM-DSC was also studied for resilin samples ( Supplementary Fig. S1 ). The non-reversing impact in thermal properties, such as the thermal contribution of water evaporation and other non-reversing transitions, are thereby eliminated for the precise identification of the two-step transitions by this technique. The results confirm that the first transitions of resilin samples occurred around 50 °C. The second transition temperatures 201, 171 and 190 °C are for pure full-length resilin, exon I and III, respectively. A similar result for the second transition temperature (175 °C) of pure exon I was also determined by local thermal analysis [9] . Therefore, the thermal transitions from the glassy to the rubbery state were related to specific regions of the protein, as indicators to monitor structural changes. 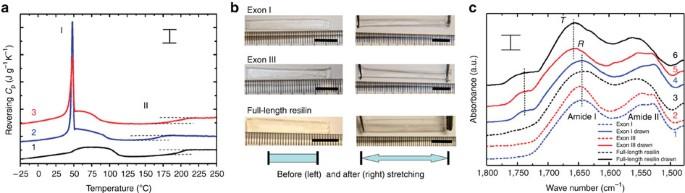Figure 2: Thermal transitions and comparative stretching studies of resilin samples. (a) Thermal transitions of resilin samples were analysed by TM-DSC for full-length resilin (1, black line), exon I (2, blue line) and exon III (3, red line), during heating at 2 K min−1. A two-step transition was indicated by TMDSC studies with step 1 in the temperature region of 30–150 °C and step 2 in 150–240 °C. The scale bar is 1 J g−1K−1. (b) Comparative analysis of resilin films for exon I, exon III and full-length resilin before (left) and after (right) stretching. The scale bar is 1 cm. (c) Selected RT-FTIR spectra in the amide I and II regions were observed for exon I (1), exon III (2), full-length resilin (3), exon I ×1.5 drawn (4), exon III ×1.5 drawn (5) and full-length resilin ×1.5 drawn (6). The scale bar is 0.5. Figure 2: Thermal transitions and comparative stretching studies of resilin samples. ( a ) Thermal transitions of resilin samples were analysed by TM-DSC for full-length resilin (1, black line), exon I (2, blue line) and exon III (3, red line), during heating at 2 K min −1 . A two-step transition was indicated by TMDSC studies with step 1 in the temperature region of 30–150 °C and step 2 in 150–240 °C. The scale bar is 1 J g −1 K −1 . ( b ) Comparative analysis of resilin films for exon I, exon III and full-length resilin before (left) and after (right) stretching. The scale bar is 1 cm. ( c ) Selected RT-FTIR spectra in the amide I and II regions were observed for exon I (1), exon III (2), full-length resilin (3), exon I ×1.5 drawn (4), exon III ×1.5 drawn (5) and full-length resilin ×1.5 drawn (6). The scale bar is 0.5. Full size image Structural characterisation in the energy inputs Real-time Fourier transform infrared spectroscopy (RT-FTIR) was used to identify the structural changes in the various resilin samples at temperatures above and below the two transitions. Amide I, II and III regions in the FTIR spectra were assessed for resilin samples from 30 to 150 °C and from 150 to 240 °C during heating at 2 K min −1 ( Fig. 3 and Supplementary Fig. S2 ). These regions were also indicated as step 1 and step 2 of resilin transitions in the TMDSC study. During the step 1 transition of full-length resilin, a strong shift in the amide II region occurred from 1,540 to 1,517 cm −1 , whereas the amide I region shifted up slightly from 1,650 to 1,658 cm −1 ( Supplementary Fig. S2a ). Absorbance in amide II is mainly due to NH in-plane bending and CN stretching vibrations and consists mostly of side chain vibrations in the protein backbone [10] . After the loss of bound water in the resilin structure, most larger side chain functional groups, such as tyrosine side chains (1,515 cm −1 ), repack and extend outward from the protein backbone to form a tighter and more ordered structure, as previously reported for silk fibroin and bovine serum albumin [10] , [11] . In addition, it has been generally agreed that the shift of peak from around 1,550 to around 1,530 cm −1 in amide II indicated a possible transition of α-helix to β-structure in the protein structure [12] , [13] . However, the relatively smaller shift in the amide I region indicated no obvious changes of secondary structures, which was also confirmed by a weak shift from 1,239 to 1,231 cm −1 in the N–H bending sensitive amide III region ( Supplementary Fig. S2d ). Therefore, this step 1 transition could be related only to the formation of a primary structure in resilin such as PPII-like conformation, which is an in-trans precursor structure prepared for the further transition of protein structures [14] , [15] . The precursor conformation has been found in many structural proteins, such as elastin, spider silk and collagen, and is believed to have an intermediate role in self-assembly [16] , [17] . However, no strong hydrogen bonds were found in the amide I region, as is the case for most precursor structures, and only a small shift was noted for a helix-enriched region around 1,658 cm −1 . In this process, the bound water is involved in promoting the formation of a precursor structure in full-length resilin. 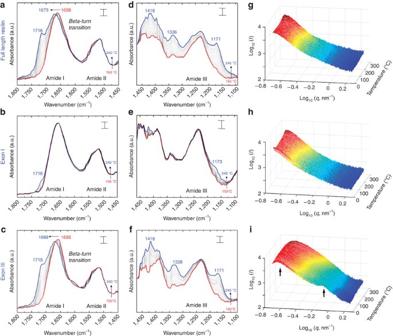Figure 3: Structure determinations of resilin samples. Selected RT-FTIR spectra in the amide I, II and III regions were analysed for full-length resilin (a,d), exon I (b,e) and exon III (c,f) during heating at 2 K min−1. Transitions were indicated as TMDSC studies for step 2 from 150 °C (red trace) to 240 °C (blue trace). The scale bar is 0.1 fora,bandc, and 0.02 ford,eandf. Temperature development of structure was also performed using SAXS, Log(I) versus log(q) data are shown for full-length resilin (g), exon I (h) and exon III (i) samples. Figure 3: Structure determinations of resilin samples. Selected RT-FTIR spectra in the amide I, II and III regions were analysed for full-length resilin ( a , d ), exon I ( b , e ) and exon III ( c , f ) during heating at 2 K min −1 . Transitions were indicated as TMDSC studies for step 2 from 150 °C (red trace) to 240 °C (blue trace). The scale bar is 0.1 for a , b and c , and 0.02 for d , e and f . Temperature development of structure was also performed using SAXS, Log(I) versus log(q) data are shown for full-length resilin ( g ), exon I ( h ) and exon III ( i ) samples. Full size image After the formation of the precursor structure in the full-length resilin with the help of bound water, there is a strong hydrogen bond-related structural transition above 201 °C ( Fig. 3a ). A peak centred at 1,716 cm −1 appeared and increased rapidly during the step 2 transition, which is due to the increase of strong –COO– stretching vibrations in the side chain groups of Asp, Glu and protein N, C-terminals in resilin [18] . At 240 °C, the 1,658 cm −1 peak in the amide I region shifted up to 1,673 cm −1 , indicating a beta-turn structural transition. A strong peak around 1,171 cm −1 also shifted and increased in the amide III region of the resilin spectrum ( Fig. 3d ). This change may be associated with the increasing stretching vibration of the C–O group in protein backbone during the transition [19] . However, compared with the step 1 transition, no obvious changes were found in the amide II region of full-length resilin during this beta-turn transition, suggesting no major macroscopic chain movement in resilin occurs in this process, as was also discussed previously for silk [10] . Similar precursor structures in step 1 transitions were demonstrated for the peptides from exon I ( Supplementary Fig. S2b and e ) and exon III ( Supplementary Fig. S2c and f ) as were observed for full-length resilin. However, a large difference in structure was found during the secondary transitions of both exons. No obvious structural transition was evident for the peptide from exon I, even when heated above 240 °C, with only a slight increase in the peak at 1,711 cm −1 ( Fig. 3b,e ). Previous studies of pro-resilin (exon I) have reported a largely unstructured protein without beta-turn conformation during heating up to 80 °C in solution [6] . In contrast, an obvious beta-turn structural transition was observed for exon III in this work, similar to that found for full-length resilin ( Fig. 3c,f ). The 1,655 cm −1 peak in the amide I region shifted to 1,669 cm −1 of the beta-turn conformation, with a strong vibration increase in the 1,715 cm −1 peak. Therefore, exon III and full-length resilin samples possess similar beta-turn transitions, compared with the unstructured exon I sample. The cooled full-length resilin films were analysed again by FTIR after being maintained at room temperature for 2 days. Partial return of the beta-turn conformation (1,673 cm −1 ) to the unstructured conformation (1,650 cm −1 ) was detected in the amide I region, and a reverse side chain peak partially shifted from 1,517 to 1,540 cm −1 in the amide II region ( Supplementary Fig. S3 ). This observation may result from atmospheric water absorbed by the resilin. When insufficient time is given for water absorption to occur, the changes are reversible. For example, no changes in the spectrum of full-length resilin were found after fast heating and cooling (>20 K min −1 ) performed from 30 to 240 °C and then back to 30 °C, indicating a reversible beta-turn transition in full-length resilin with controlled energy input and release. In addition, to identify the persistence of the beta-turn transition by input of mechanical energy, all unheated full-length resilin, exon I and exon III films were stretched up to 1.5 times from the original length before breaking and FTIR spectra of resilin films were collected before and after the stretching ( Fig. 2b,c ). Beta turns increased for both full-length and exon III resilin samples after the stretching, whereas exon I did not show a significant change, consistent with the data above. To further understand the material functions of both exons in native resilin, we also used an atomic force microscopy (AFM) to measure the nanomechanical properties at the molecule level, similar to conventional compression tests [3] , [20] . Based on force-distance curves by AFM ( Supplementary Fig. S4 ), exon I exhibited >90% resilience, compared with 65% resilience for exon III, indicating exon I offered similar material functions to the full-length protein and contributes critical elasticity for the native resilin. In nature, energy input and release from resilin can be accomplished by extensional forces during the movement of insect muscles, versus the use of heat in the current report. According to thermodynamic theory of rubber elasticity in polymer physics [21] , the change in temperature directly relates to the change of extensional force in polymer materials as follows: where L is the material length, U is the internal energy of the material, and f U and f S are the energy and entropy contributions to the total extensional force ( f ) at the temperature ( T ). For an ideal elastomer, the internal energy change, (∂ U /∂ L ) T is nearly zero compared with the second term. Thus, the force and the temperature measured at constant length have an almost linear correlation for elastomeric materials, thereby allowing comparisons between temperature-induced transitions versus mechanical force inputs in biological systems. We demonstrated the beta-turn transition by FTIR with slow heating to 240 °C, but this high or overloaded thermal energy input to resilin resulted in a partially permanent non-elastic transformation. This feature is analogous to an overloaded elastic spring in the case of mechanical stretching, which goes beyond Hooke's Law elastic regime. In nature, the energy released and restored in resilin occurs instantly, with precise loading controlled via muscles by the insect, so the resilin can endure extension and retraction over millions of cycles over the lifetime of the animals. Synchrotron RT small-angle X-ray scattering (SAXS) studies were carried out to further identify the structural changes during heating from 30 to 265 °C at 2 K min −1 for full-length resilin ( Fig. 3g ), exon I ( Fig. 3h ) and exon III ( Fig. 3i ) samples. The full-length resilin and unstructured exon I in Fig. 3g,h , respectively, had no obvious small angle peak over the investigated temperature range, suggesting no large-scale periodic structure can form in these samples. However, clear small angle peaks were observed in the exon III sample ( Fig. 3i ), with a major low q peak around 0.18–0.31 nm −1 , and a weak high q peak around 0.78–1.19 nm −1 . The peak from the small angle X-ray pattern indicates an alternating periodic structure with a relationship q =2π/ d , where q is q -vector ( q =4πsinθ/λ, for θ the half-scattering angle, and λ=0.137 nm) and d (D-spacing) is the periodic distance between long-range ordered structures in the material. To better understand this process, the major low q SAXS peak was analysed as to the peak position as a function of temperature, and these data are shown in Supplementary Fig. S5a , as well as a slow-frame 'movie' included as Supplementary Movie 1 . During the step 1 transition from 30 to 90 °C, the D-spacing value for periodic structures of exon III peptides first increased in the presence of bound water molecules from ~29 nm to at least ~35 nm (observable maximum up to the region covered by the beam stop), then it decreased back to ~29 nm, probably related to the loss of bound water. The D-spacing value remains stable from 90 to 205 °C until passing through the step 2 transition. After the second transition temperature around 200 °C, the peak position continuously decreased from ~29 to ~25 nm at 250 °C, which may be related to the beta-turn transition in the molecular level observed by FTIR studies in the paper. The high q SAXS peaks (with D-spacing between 5.3–8.1 nm) are hard to precisely interpret due to the noise, although they may be possibly related to periodic structures of single or several exon III molecules. To understand whether there are significant chemical changes in the protein samples during the thermal treatments, we also performed SDS–polyacrylamide gel electrophoresis studies for exon I, exon III, and full-length resilin proteins treated at different temperatures up to 200 °C. The results demonstrated that all protein samples are generally stable without significant molecular weight change after heating to different temperatures, indicating the proteins have not changed primary structures ( Supplementary Fig. S6 ). Primary sequence analysis The primary amino-acid sequence of full-length resilin was analysed for predictions of disordered regions, secondary structure and hydrophobicity. The structures, particularly in exon I, exhibited a highly flexible conformation with overall structural disorder ( Supplementary Fig. S7 ), which is a fundamental requirement for elastomeric function [22] . Further predictions suggested a high degree of random coil and the presence of beta turns in exon I and III, and an ordered structure of alpha helix in the part of exon II ( Supplementary Fig. S8 ). Beta turns are believed to be critical for energy storage and release in elastic proteins [6] . The examination of the primary sequence of resilin shows hydrophilic blocks or domains ( Fig. 1d ), suggesting strong interactions between bound water and the side chains of resilin in the self-assembly process. The hydrophilic properties of resilin may help form a homogenous plasticized bound water–protein system, resulting in additional chain mobility at lower temperature. Surface morphology and structure transitions Exon I encodes a peptide with more hydrophilic blocks with more disordered structures than exon III, behaving like a more flexible structure with extended chains in water. On the basis of backbone hydration and hydrogen bonding, exon I-encoding regions begin to self-aggregate into organized fibrillar structures. After the loss of bound water upon heating, the exon I peptide condenses and self-assembles into a tighter and more organized aligned globules ( Fig. 4a ). The interpretation of this behaviour is supported by AFM and scanning electron microscopy (SEM). The surface morphology of resilin samples before and immediately after thermal treatments showed nanostructure changes at the thermal transitions ( Fig. 4 ; Supplementary Fig. S9 ). Both untreated and thermally treated exon I peptide showed similar surface morphology with nanoscale inhomogeneous patterns [9] , with the particle size slightly compressed or shrunken into tighter globules from ~30 to ~20 nm in diameter after thermal treatment ( Fig. 4a ). This change in morphology is consistent with the observation of no strong structural transitions for exon I during thermal treatment. 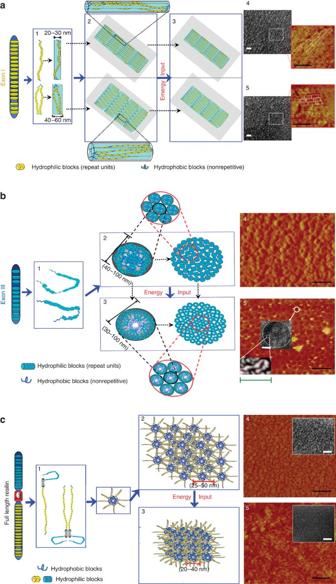Figure 4: Self-assembly mechanism of resilin proteins. (a) Model of chain folding, fibrillar structure formation and physical stress for exon I. (1) Possible chain folding intra- and inter-molecular schemes. (2) Fibril assembly with larger-chain hydrophilic blocks in contact with the surrounding aqueous solution. (3) The assembly process upon heating and alignment of fibrils and interactions promoted by physical stress. To fully understand the nanostructure changes in the thermal transitions, the surface morphology of exon I was observed in AFM phase images and by SEM before (4) and right after (5) thermal treatments. The black scale bar is 200 nm and the white is 30 nm. (b) Model of chain folding, micelle and globule formation and physical stress for exon III. (1) Possible chain folding intra- and inter-molecular schemes. (2) Micelle and globule assembly driven by hydrophilic-hydrophobic multiblock co-polymers with a larger hydrophobic block at the middle of the chain, resulting in the formation of the hydrophobic core of irregular sized globular proteins. (3) The assembly process upon heating and alignment of globules with ordered, water-excluding, core-containing micelles. The surface morphology of exon III peptides were also observed in AFM phase images and by SEM before (4) and right after (5) thermal treatments. The black scale bar is 200 nm, the white is 30 nm and the green is 5.5 nm. (c) Proposed model of resilin elasticity in the process of energy input and release. (1) Possible chain folding intra- and inter-molecular schemes. (2) Structure assembly and relaxed network driven by hydrophilic–hydrophobic–hydrophilic polymers to form water-swollen structures with irregular sized micelles crosslinked by fibrils. (3) The assembly process upon heating and tighter elastic network after energy input. The surface morphology of full-length resilin was observed in the AFM phase images and by SEM before (4) and right after (5) thermal treatments. The black scale bar is 200 nm and the white is 30 nm. Figure 4: Self-assembly mechanism of resilin proteins. ( a ) Model of chain folding, fibrillar structure formation and physical stress for exon I. (1) Possible chain folding intra- and inter-molecular schemes. (2) Fibril assembly with larger-chain hydrophilic blocks in contact with the surrounding aqueous solution. (3) The assembly process upon heating and alignment of fibrils and interactions promoted by physical stress. To fully understand the nanostructure changes in the thermal transitions, the surface morphology of exon I was observed in AFM phase images and by SEM before (4) and right after (5) thermal treatments. The black scale bar is 200 nm and the white is 30 nm. ( b ) Model of chain folding, micelle and globule formation and physical stress for exon III. (1) Possible chain folding intra- and inter-molecular schemes. (2) Micelle and globule assembly driven by hydrophilic-hydrophobic multiblock co-polymers with a larger hydrophobic block at the middle of the chain, resulting in the formation of the hydrophobic core of irregular sized globular proteins. (3) The assembly process upon heating and alignment of globules with ordered, water-excluding, core-containing micelles. The surface morphology of exon III peptides were also observed in AFM phase images and by SEM before (4) and right after (5) thermal treatments. The black scale bar is 200 nm, the white is 30 nm and the green is 5.5 nm. ( c ) Proposed model of resilin elasticity in the process of energy input and release. (1) Possible chain folding intra- and inter-molecular schemes. (2) Structure assembly and relaxed network driven by hydrophilic–hydrophobic–hydrophilic polymers to form water-swollen structures with irregular sized micelles crosslinked by fibrils. (3) The assembly process upon heating and tighter elastic network after energy input. The surface morphology of full-length resilin was observed in the AFM phase images and by SEM before (4) and right after (5) thermal treatments. The black scale bar is 200 nm and the white is 30 nm. Full size image The exon III-encoding peptide is a pattern of several internal hydrophobic and hydrophilic domains with a larger hydrophobic block in the middle chain of protein, suggesting the possibility for formation of micellar structures in water ( Fig. 4b ). The hydration of hydrophilic blocks initially helps form a more extended chain structure until the hydrophobic regions begin to assemble and organize into micelles, resulting in the formation of the hydrophobic core of irregularly sized globules depending on chain folding and hydrophobic interactions. During the thermal transitions described above, exon III peptide self-aggregates upon heating to ordered, water-excluding, core-containing micelles. This significant change in exon III peptide nanostructure was also demonstrated in morphology studies before and after thermal treatment ( Fig. 4b ). The untreated sample showed inhomogeneous nanoparticle patterns with sizes around 40–100 nm. However, larger and more homogenous nanoporous patterns were observed on the surface, with pore diameters around 30–100 nm after the beta-turn transition discussed above. We also performed optical transforms (based on the Fast Fourier Transform algorithm) of large-scale AFM images from Fig. 4b to confirm this, as shown in Supplemental Fig. 5b . In some cases, exon III spheres that were not completely transferred by heat energy input still remained and could be seen on the AFM pictures ( Supplemental Fig. 5b , arrows). The existence of this beta-turn structural conversion is often experimentally found to be critical for the elasticity of protein elastomers and believed to function in energy storage and release [6] , [23] . More recently, the mechanical stretching simulations provide insight into the nanoscale deformation mechanisms, suggesting the importance of beta-turn structural change at the molecular level for energy storage and release in spider dragline silk [24] , [25] . Molecular mechanism of resilin elasticity Taken together, and with additional interactions of exon II peptide ( Fig. 1 ; Supplementary Figs S7 and S8 ), including more ordered and hydrophobic structures, the model of resilin assembly suggests that the protein acts as a hydrophilic–hydrophobic–hydrophilic polymer to form water-swollen structures with irregular sized micelles ( Fig. 4c ). After the loss of water and transitions upon heating, the full-length resilin self-aggregates to form a nonhomogeneous nanoporous pattern with island-like networks, with pore sizes around 20–40 nm, which were observed to be a tightly packed irregular nanoparticles with a size of 25–50 nm before thermal treatment ( Fig. 4c ). Hydrophobic blocks direct the folding and formation of micelles in the process of assembly. The physical stress may induce subtle interactions among the protein domains to self-organize into more functional nanostructures by limited hydrophobic interactions after the loss of water upon heating. Based on the properties of resilin summarized in Table 1 , full-length resilin is considered uncrystallizable but able to perform a beta-turn structural transition. Such a transition is mainly contributed by exon III peptide with its long-range periodic structure. The structural repacking for energy storage was indicated by the changes in the protein during thermal treatment. Exon III is the 'hard' segment in the resilin protein with only around 65% resilience [20] . However, the unstructured and non-crystallizable properties of exon I contribute the super elasticity of the resilin protein, without a strong structural transition shown. Exon I tends to be the 'soft' segment and possess resilience of >90% [3] , [7] . The resilin network can be biochemically crosslinked between tyrosine residues, which help to construct a similar thermoplastic elastomeric polymer network [26] , [27] . In addition, transmembrane segments of full-length resilin were predicted ( Fig. 1e ). Exon I is predicted to be located outside the cell membranes, and have the role of a supporting network with its super elasticity, whereas exon III is thought to be located inside the cell membrane, suggesting it is a perfect candidate for storing and releasing energy in insect tissue. Therefore, we propose a molecular mechanism of resilin elasticity. The resilin network remains in a relaxed state without beta-turn conformations before physical stress. Upon energy input, such as via mechanical stress or thermal treatment, exon I regions respond immediately because of the super elasticity and release the energy to the exon III regions. The exon III regions of the protein transform to a more ordered beta-turn structure. These changes result in elastic energy conversion with high efficiency during energy input such as mechanical stress. After the energy is removed or reduced, exon III regions of the protein recover to an unstructured conformation and release the stored potential energy to the elastic network of exon I protein regions, resulting in the jumping or flying movement of insects. In these contraction/extension cycles, insects in nature must control the structural changes and the energy conversion process with resilin within their physiology environments over their entire lifetime. Thus, water content, protein fatigue and biochemical factors in the insect all have an important role in the rapid deformation of resilin in vivo with controllable energy input and release. Table 1 Properties of resilin samples. Full size table In contrast to other elastic proteins such as elastin or elastin-like proteins with hydrophobic blocks (VPGVG) n [6] , many models including ordered beta-spiral, sliding beta-turn and random network, have been constructed to discuss how beta-turn-related configurations contribute to protein structure and function, emphasising beta turns of natural elastic proteins as fundamental units of the structure and elasticity as the major stable conformations in protein chains [6] , [28] . Nanoscale features of biological materials are crucial to achieve the associated mechanical properties. Recent computational investigations of the silk nanostructure revealed the mechanistic interplay of the two constitutive phase of silk, semi-amorphous regions and highly organized beta-sheet nanocrystals, as well as the effect of structural changes on the overall mechanical behaviour, providing us with a powerful alternative to the traditional engineering top-down approach of shaping materials to obtain specific properties and enable the bottom-up design of complex materials [24] , [25] . Another example to demonstrate the importance of structure changes for protein elastomer systems is the Busycon egg capsule wall, which has been well known to have high extensibility, durability and shock-absorbing capability. Thermomechanical and structural analyses have indicated that the long-range elasticity of the capsules is associated with the internal energy arising from the fully reversible structural α-helix↔β-sheet transition of egg capsule proteins during extension [29] . In addition, external factors might be correlated to the elastic moduli of the protein elastomer systems [30] . The process described here illustrates the unique combination of protein sequence domains and physical chemistry in the dynamic function of resilin proteins. We have focused on the solid state structures of resilin, which contain bound water after drying. The results revealed a β-turn transition as a key to the elasticity mechanism for native resilin, which could be useful for explaining other elastic proteins in nature. During the glass transition of the proteins, their molecular chains obtain enough thermal energy for movement from restricted local vibrations to long-range rotational motion, which promotes self-assembly to a preferred ordered structure with lower-molar potential energy. The elucidation of this mechanism also suggests polymer designs and processing in aqueous environments as a route to obtain such desired functional elastomeric properties, leading to new opportunities in biomimetics, biomaterials and tissue engineering, all within a green chemistry context. Protein materials and sequence analysis Cloning, expression and purification of recombinant resilin proteins have been done as described previously [7] . A final 1% aqueous solution of resilin samples were cast in polystyrene Petri dishes to generate films with a thickness of 10–20 μm without any treatments. Films were placed in a vacuum oven at room temperature for 1 day to remove surface moisture. The films containing 8–15% bound water, determined by thermogravimetric analysis [31] , were completely unstructured and non-crystalline before thermal treatment. Sequence analysis was performed for resilin hydrophobicity, with a window of 9 used as reported previously [32] . Disordered regions of a protein chain were predicted based on its amino-acid sequence in the PrDOS server ( http://prdos.hgc.jp ) [33] . Transmembrane regions of resilin protein chain were also predicted based on its amino-acid sequence in the ANTHEPROT server ( http://antheprot-pbil.ibcp.fr ) [34] . Secondary structure of resilin was further analysed as reported [35] . Differential scanning calorimetry (DSC) About 3 mg resilin samples were encapsulated in aluminium pans and heated in a TA Instruments Q100 DSC with a dry nitrogen gas flow of 50 ml min −1 , and equipped with a refrigerated cooling system. The instrument was calibrated for empty cell baseline with indium for heat flow and temperature. Sapphire reference standards were also used for calibration of the heat capacity. By a DSC measurement with a constant applied heating rate, we obtain the total heat capacity based on total heat flow, which consists of both the reversing and non-reversing components as follows: where mC p is the heat capacity of a sample of mass, m; K ″ is a calibration constant; HF is heat flow; and q is the underlying heating rate. TM-DSC measurements were performed at 2 K min −1 with a modulation period of 60 s and temperature amplitudes of 0.318 K. The same empty Al reference pan was used in all runs, and all empty sample pans before loading samples were selected to be the same weight. By adding a sinusoidal modulation on the conventional constant heating or absolute isotherms [10] , TMDSC changes the heater temperature T ( t ) by: where T 0 is the initial temperature, q is the underlying heating rate, A is the corresponding oscillation amplitude and the frequency of oscillation is with p being the period in seconds and θ is the phase shift with respect to the reference. In TMDSC the 'reversing heat flow' is measured, a term representing a heat effect, which can be reversed within the temperature range of the modulation [10] , [31] , [36] . Therefore, the 'reversing heat capacity' can be calculated from: where mC p is the heat capacity of a sample of mass, m , and specific heat capacity, C p ; C s is heat capacity of the sample pan and C r is the heat capacity of an empty reference pan; Δ C cell is the cell asymmetry correction, which can be determined by running a series of empty pans with various mass differences compared with the reference [10] . On the right hand side of equation (4), A T is the amplitude of temperature difference between sample and reference; A is the sample temperature modulation amplitude; K is Newton's law calibration constant, which is independent of modulation frequency and reference; A HF is the heat flow amplitude and K ′ is a calibration constant at each individual temperature provided the same experimental conditions are maintained to assure the same heat transfer (for example, same reference, same modulation frequency). If the heat capacity is reversing, equations (2) and (4) give the same result; if not, the difference between (2) and (4) gives the non-reversing heat capacity component. All DSC measurement consisted of three runs as described in our earlier work [10] , [31] . The first run is empty Al sample pan versus empty Al reference pan to obtain the cell asymmetry and baseline correction. The second run is sapphire standard versus empty Al reference pan to calibrate heat flow amplitude according to standard equations as published previously [10] , [31] . The third run is sample versus empty Al reference pan. The same empty Al reference pan was used in all the runs, and all the Al sample pans were kept the same in weight. Fourier transform infrared spectroscopy (FTIR) The resilin samples were put into an optical microscopy hot stage (Mettler, FP90) as free-standing films (no IR transparent substrate was used) and examined in transmission mode. This hot stage was then placed under an IMV-4000 multi-channel FTIR microscopic spectrometer (Jasco, Japan) with a liquid nitrogen cooled mercury cadmium telluride detector. The analysis was performed in transmission mode using the microscope. The temperature in the heating holder was monitored with the central processor of the hot stage and was calibrated with a thermocouple before the experiments. The instrument was sealed and continuously purged by nitrogen gas to prevent oxidative chemical changes of samples during the studies. The aperture to give the best signal-to-noise ratio was 10 μm. For each measurement, 128 scans were co-added and Fourier transformed using a Genzel-Happ apodization function to yield spectra with a nominal resolution of 4 cm −1 . The frequency ranged from 400 to 4,000 cm −1 . To identify structures of protein samples from the absorption spectra, we obtained the positions of the absorption band maxima from Fourier self-deconvolution performed by using the Opus 5.0 software (Bruker) as described previously [37] . The assignment of adsorption peaks in amide I band is generally agreed with all of peptides [38] , [39] , as well as resilin-related proteins [2] , [20] : the broad peak centered at 1,640–1,660 cm −1 to random coil or helical conformation, or both; the peak from 1,615 to 1,640 cm −1 to β-sheet conformation; and the peak from 1,660 to 1,695 cm −1 to β-turn conformation. All figures presented in this work show only raw (unsmoothed) absorption data corrected by background subtraction. Synchrotron X-ray scattering analysis Time-resolved SAXS experiments were conducted at Brookhaven National Laboratory, National Synchrotron Light Source beam line X27C with a wavelength of 0.1371 nm. One-dimensional position-sensitive gas-filled wire detectors (Braun) were used to collect the scattered intensity. Silver behenate and Al 2 O 3 standard reference powders were used to calibrate the q -vector. The samples were heated from 30 to 265 °C with a heating rate of 2 °C min −1 , and the X-ray intensity was accumulated every minute (that is, with temperature interval of two degrees) until the end of the thermal ramping. The powder-like resilin samples were encapsulated in high-temperature Kapton tape and heated inside a temperature-controlled hot stage (Mettler). The intensity was monitored upstream and downstream of the sample and the intensity, I ( q ), was corrected for sample absorption, changes in incident beam intensity with time, and Kapton tape background. Intensity data were averaged in temperature space over a sliding window with a width of 6 °C (corresponding to averaging 3 min of data collection). The temperature is reported as the midpoint of each window. The location of the intensity peak maximum was determined at all temperatures by fitting either the intensity versus q , or log (intensity) versus log ( q ), curves with a polynomial function. Atomic force microscopy (AFM) All imaging was performed in tapping mode on a Dimension 3100 Scanning Probe Microscope with Nanoscope V controllers (Digital Instruments, Santa Barbara, CA, USA) and equipped with rotated tapping-mode etched silicon probes (Nanodevices, Santa Barbara, CA, USA). Resilin solution samples were cast on silicon surfaces to form thin films before thermal treatment. AFM observations were performed in air at room temperature using a 225-μm long silicon cantilever with a spring constant of 3 N m −1 . Calibration of the cantilever tip-convolution effect was carried out to obtain the true dimensions of objects by previously reported methods [38] . Scanning electron microscopy (SEM) SEM was used to assess additional morphological characterisation of the protein samples. The experiments were performed using a Zeiss 55VP System (Oberkochen, Germany, at Harvard University Center for Nanoscale Systems, Cambridge, MA). Proteins were first dried on a silicon chip in a closed container at room temperature before thermal treatments. Nanomechanical testing Measurements of elastic modulus and elasticity (resilience %) on the protein samples were conducted using AFM operated in force mode. Force-distance curves for each sample were measured at least 10 times in each different region, and s.d. determined. To clearly demonstrate the difference in resilience, the deflection values were normalized to between 0 and 100 nm. The elasticity (resilience) calculated is defined as the energy recovered after removal of the stress, divided by the total energy of deformation. The energy of deformation/recovery is given by converting force displacement curves into force-penetration/retraction curves, and calculating the ratio of the areas under the penetration and retraction curves [3] , [7] , [20] , [40] . The values were averaged based on measurements of 20 points on the surface of each sample. The calculation of elasticity (resilience) has been discussed in detail for elastic resilin proteins in our previous studies [7] , [20] , [39] . How to cite this article: Qin, G. et al . Mechanism of resilin elasticity. Nat. Commun. 3:1003 doi: 10.1038/ncomms2004 (2012).